Scalable fabrication of high-power graphene micro-supercapacitors for flexible and on-chip energy storage The rapid development of miniaturized electronic devices has increased the demand for compact on-chip energy storage. Microscale supercapacitors have great potential to complement or replace batteries and electrolytic capacitors in a variety of applications. However, conventional micro-fabrication techniques have proven to be cumbersome in building cost-effective micro-devices, thus limiting their widespread application. Here we demonstrate a scalable fabrication of graphene micro-supercapacitors over large areas by direct laser writing on graphite oxide films using a standard LightScribe DVD burner. More than 100 micro-supercapacitors can be produced on a single disc in 30 min or less. The devices are built on flexible substrates for flexible electronics and on-chip uses that can be integrated with MEMS or CMOS in a single chip. Remarkably, miniaturizing the devices to the microscale results in enhanced charge-storage capacity and rate capability. These micro-supercapacitors demonstrate a power density of ~200 W cm −3 , which is among the highest values achieved for any supercapacitor. The current trend with portable electronics lies in continuous miniaturization, while enhancing the functionality and reliability of existing components. However, the integration of energy-storage units—that is, batteries and supercapacitors—with electronic circuits is challenging, and often limits the miniaturization of the entire system. This is because the necessary energy-storage components scale down poorly in size and are not well suited to the planar geometries of most integrated fabrication processes. Progress in micro-fabrication technology has enabled on-chip micro-supercapacitors in an interdigitated planar form in contrast to the conventional sandwich structure–the latter being incompatible with integrated circuits [1] . Among the most desirable properties of a micro-supercapacitor, high-power density, high-rate capability and especially high-frequency response are crucial for future applications [2] , [3] . From a materials perspective, carbon is earth abundant and inexpensive; hence, many nanostructured carbon-based materials have been studied for use in electric double-layer (EDL) micro-supercapacitors, including activated carbons [4] , carbon nanotubes [5] , carbide-derived carbons [1] , [6] and onion-like carbon [2] . In addition, transition metal oxides such as ruthenium oxide [7] and manganese oxide [8] , and conducting polymers such as polypyrrole [9] and polyaniline [10] have been used as materials for pseudo-capacitive micro-supercapacitors. Among all the previous examples, only onion-like carbon has produced a micro-supercapacitor with ultrahigh-power handling with an RC time constant of only 26 ms (ref. 2 ). However, the high-temperature processing of onion-like carbon and the scalability problems of the fabrication technique limit the potential of these devices. Graphene, a two-dimensional carbon sheet with monoatomic layer thickness, offers great potential for energy storage [11] , [12] , [13] . With its high theoretical surface area (2630, m 2 g −1 ) and electrical conductivity, graphene could produce supercapacitors with ultrahigh power. We [11] and others [13] , [14] , [15] have developed thin-film graphene supercapacitors that demonstrated high-power performance with superior frequency response. Although promising, the sandwich structure of these supercapacitors limits their integration into electronic circuits. Yoo et al. [16] observed a marked increase in the specific capacitance of graphene supercapacitors when made in a planar structure. Later, this research group developed a process for the direct writing of planar graphene micro-supercapacitors through the laser reduction and pattering of hydrated graphite oxide (GO) films [17] . Having discovered that hydrated GO is simultaneously a good ionic conductor and an electrical insulator, they used hydrated GO as both the separator and electrolyte to simplify the fabrication of the device. Although this fabrication technique is promising, the poor frequency response and the large internal resistance (6.5 kΩ) of the as-made devices are not adequate for practical applications. Most recently, Beidaghi et al. [3] reported graphene/CNT composite micro-supercapacitors using a combination of micro-fabrication techniques and electrostatic spray deposition. They measured a high volumetric capacitance with an RC time constant as low as 4.8 ms. However, all the fabrication methods reported so far involve conventional lithographic techniques or employ masks for the definition of patterns on substrates. Unfortunately, these methods are awkward for building cost-effective devices for commercial applications. Therefore, the challenge is to develop a simple, inexpensive high-throughput lithographic technique that does not require masks, additional processing or sophisticated operation while producing high-performance micro-devices. In consideration of the problems described above, we report on the direct fabrication of interdigitated graphene micro-supercapacitors using a consumer-grade LightScribe DVD burner. This process is readily scalable, and the devices can be fabricated on large substrates at a fraction of the cost of traditional micro-fabrication methods. The produced devices are extremely thin, of all-solid state and are completely flexible. We also describe the first experimental demonstration of an all-solid-state micro-supercapacitor using an ionogel electrolyte that allows the operation of the device at a voltage window of 2.5 V compared with 1 V for traditional hydrogel-polymer electrolytes. Recently, considerable efforts have been made for the fabrication of flexible micro-supercapacitors for the emerging electronics industry. However, none of these configurations have been shown to be suitable for flexible energy storage. The micro-supercapacitors demonstrated here show exceptional electrochemical stability under different bending and twisting conditions. These microscale supercapacitors can also be fabricated on-chip for the next generation of CMOS applications. Moreover, by varying the dimensions of the interdigitated micro-electrodes, it is possible to control the energy and power handling of these devices. These supercapacitors exhibit an ultrahigh power of ~200 W cm −3 and excellent frequency response with an RC time constant of only 19 ms. Fabrication of laser-scribed graphene micro-supercapacitors LightScribe is a direct-to-disc labelling technology that burns text and graphics onto the surface of a CD or DVD using a laser inside the drive [18] . To make these labels, the surface of the disc is coated with a reactive dye that changes colour on exposure to the laser light. Instead of printing on this specialized coating, our approach is to coat the disc with a film of GO, which then can be directly printed upon. The process is schematically illustrated in Fig. 1 . Circuits designed on a computer can be patterned onto the DVD disc, which is now coated with a film of GO. We [19] and others [20] originally found an unusual photo-thermal effect in which GO absorbs high-intensity light and is converted into graphene. By using the precision of a laser, the drive renders the computer-designed pattern onto the GO film to produce the desired graphene circuits [21] . In this way, interdigitated graphene electrodes can be readily LightScribed on the disc, as shown in Fig. 1a . This form of graphene is called laser-scribed graphene (LSG). With its nearly insulating properties, GO serves as a good separator between the positive and negative graphene interdigitated electrodes [17] . These graphene circuits can thus be directly used as planar micro-supercapacitors after receiving an electrolyte overcoat, Fig. 1b . Unlike conventional micro-fabrication methods, this direct ‘writing’ technique does not require masks, expensive materials, post-processing or clean room operations. Furthermore, the technique is cost effective and readily scalable. For example, using the design we chose for this work, 112 micro-supercapacitors can be produced on a single piece of GO deposited on a DVD disc, Fig. 1d (see also Supplementary Fig. S1 ). Interdigitated electrodes can be precisely patterned with a lateral spatial resolution of ~20 μm using LightScribe, Supplementary Fig. S2 . This technique is thus appropriate for the fabrication of high-resolution micro-supercapacitors, taking into account that the interdigitated electrodes made with conventional micro-fabrication techniques are usually on the order of ~100 μm (with the exception of refs 1 , 6 ). 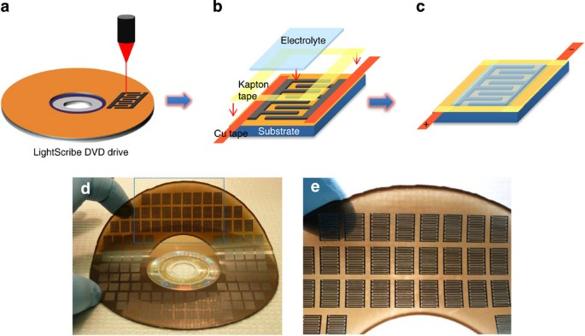Figure 1: Fabrication of LSG-MSC (a–c) Schematic diagram showing the fabrication process for an LSG micro-supercapacitor. A GO film supported on a PET sheet is placed on a DVD media disc. The disc is inserted into a LightScribe DVD drive and a computer-designed circuit is etched onto the film. The laser inside the drive converts the golden-brown GO into black LSG at precise locations to produce interdigitated graphene circuits (a). Copper tape is applied along the edges to improve the electrical contacts, and the interdigitated area is defined by polyimide (Kapton) tape (b). An electrolyte overcoat is then added to create a planar micro-supercapacitor (c). (d,e) This technique has the potential for the direct writing of micro-devices with high areal density. More than 100 micro-devices can be produced on a single run. The micro-devices are completely flexible and can be produced on virtually any substrate. Figure 1: Fabrication of LSG-MSC ( a – c ) Schematic diagram showing the fabrication process for an LSG micro-supercapacitor. A GO film supported on a PET sheet is placed on a DVD media disc. The disc is inserted into a LightScribe DVD drive and a computer-designed circuit is etched onto the film. The laser inside the drive converts the golden-brown GO into black LSG at precise locations to produce interdigitated graphene circuits ( a ). Copper tape is applied along the edges to improve the electrical contacts, and the interdigitated area is defined by polyimide (Kapton) tape ( b ). An electrolyte overcoat is then added to create a planar micro-supercapacitor ( c ). ( d , e ) This technique has the potential for the direct writing of micro-devices with high areal density. More than 100 micro-devices can be produced on a single run. The micro-devices are completely flexible and can be produced on virtually any substrate. Full size image Characterization of LSG micro-devices The laser-scribing process is associated with significant changes in the optical properties, the electrical properties and the structure of the film. For example, GO changes from a golden-brown colour to black, which is a direct impact of the reduction of GO into graphene. 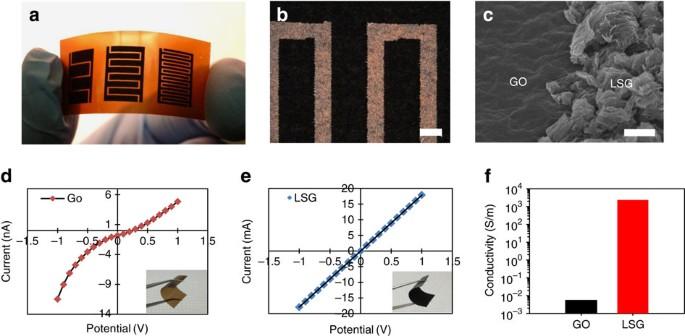Figure 2: Characterization of LSG micro-devices (a) A digital photograph of the laser-scribed micro-devices with 4 (LSG-MSC4), 8 (LSG-MSC8) and 16 interdigitated electrodes (LSG-MSC16). (b) An optical microscope image of LSG-MSC16shows interdigitated fingers with 150-μm spacings. The dark area corresponds to LSG and the light area is GO. Scale bar, 200 μm. (c) A tilted-view (45°) SEM image shows the direct reduction and expansion of the GO film after exposure to the laser beam. Scale bar, 10 μm. (d) and (e) show the I–V curves of GO and LSG, respectively. LSG exhibits a current enhanced by about 6 orders of magnitude, confirming the change from nearly insulating GO to conducting LSG. (f) A comparison of electrical conductivity values for GO and LSG. Figure 2a shows a photograph of the as-prepared LSG micro-supercapacitors (LSG-MSC). A micro-device was constructed with 16 interdigitated microelectrodes— 8 positive and 8 negative electrodes. An optical microscope image shows a well-defined pattern with no short circuits between the microelectrodes; Fig. 2b shows the expansion of the film when treated with the laser, thus enabling full access to the electrode surface that is essential for charging the electrodes (see also Supplementary Fig. S3 ). Analysis of the cross-section of the micro-device reveals a thickness of 7.6 μm. For comparison, I–V tests were carried out for both GO and LSG as shown in Fig. 2d , respectively. The GO film exhibits nonlinear and slightly asymmetric behaviour, with a differential conductivity value ranging from 8.07 × 10 −4 to 5.42 × 10 −3 S m −1 depending on the gate voltage. Reducing GO within the DVD burner results in a linear I–V curve associated with a significant increase in the film conductivity to 2.35 × 10 3 S m −1 as calculated for the LSG, Fig. 2f . Because of its high electrical conductivity and exceptionally high surface area of over 1500, m 2 g −1 , LSG can serve as both the electrode material and current collector [11] . This simplifies the fabrication process and results in cost-effective micro-supercapacitors. Figure 2: Characterization of LSG micro-devices ( a ) A digital photograph of the laser-scribed micro-devices with 4 (LSG-MSC 4 ), 8 (LSG-MSC 8 ) and 16 interdigitated electrodes (LSG-MSC 16 ). ( b ) An optical microscope image of LSG-MSC 16 shows interdigitated fingers with 150-μm spacings. The dark area corresponds to LSG and the light area is GO. Scale bar, 200 μm. ( c ) A tilted-view (45°) SEM image shows the direct reduction and expansion of the GO film after exposure to the laser beam. Scale bar, 10 μm. ( d ) and ( e ) show the I–V curves of GO and LSG, respectively. LSG exhibits a current enhanced by about 6 orders of magnitude, confirming the change from nearly insulating GO to conducting LSG. ( f ) A comparison of electrical conductivity values for GO and LSG. Full size image Evaluation of the performance of LSG-MSC To understand the role of the micro-scale architecture of the device on its electrochemical properties, different configurations were designed and tested. Micro-supercapacitors with 4 (MSC4), 8 (MSC8) and 16 (MSC16) interdigitated microelectrodes were constructed and their electrochemical performance at 1,000, 5,000 and 10,000 mV s −1 tested, as shown in Fig. 3a–c . Here, a hydrogel-polymer electrolyte, poly(vinyl alcohol) (PVA)-H 2 SO 4 , was used to fabricate the all-solid-state LSG-MSCs. A sandwich-type LSG supercapacitor was also tested for comparison ( Supplementary Fig. S4 ). The cyclic voltammetry (CV) profiles are all rectangular in shape, confirming the formation of an efficient EDL capacitor and fast charge propagation within the electrodes. Even at an ultrafast scan rate of 10,000 mV s −1 , the CV remains rectangular in shape, indicating the high-power capability of this micro-supercapacitor (see also Supplementary Fig. S5 ). Recently, it has been shown that the volumetric and areal capacitances give a more accurate picture of the true performance of a supercapacitor compared with gravimetric values [22] , [23] . This is even more relevant in the case of micro-devices, as the mass of the active material is very small. Therefore, we have calculated the specific capacitance of the micro-devices based on the volume of the stack. This includes the combined volume of the active material, current collector and the gap between the electrodes. The stack capacitances of the different micro-supercapacitors as a function of the scan rate are shown in Fig. 3d . Interestingly, the micro-devices show higher capacitance when using the interdigitated structure as opposed to the sandwich structure. Furthermore, the more the interdigitated electrodes per unit area, the more the power and energy that can be extracted from the micro-devices. This can be explained by the unique porous network structure of the LSG electrodes, which helps minimize the pathway for ion diffusion from the electrolyte to the electrode material. Moreover, the micro-scale architecture of the devices results in a significant reduction of the mean ionic diffusion pathway between two microelectrodes. This effect becomes even more pronounced when increasing the number of interdigitated electrodes per unit area (see also Supplementary Figs S6–S8 ). This allows for maximizing the available electrochemical surface area and results in the increased capacitance and the fast charge/discharge rates observed with the micro-devices. These conclusions are confirmed by the galvanostatic charge/discharge curves, Fig. 3e . Note that all the micro-devices, regardless of whether they possess 4, 8 or 16 interdigitated electrodes, show nearly ideal triangular charge/discharge curves obtained at an ultrahigh current density of 1.684 × 10 4 mA cm −3 . The voltage drop at the beginning of each discharge curve, known as the iR drop, is a measure of the overall resistance of the device, and as its value is proportional to the discharge current, the small iR drop shown in Fig. 3e at a high discharge current indicates a very low resistance for all of the micro-supercapacitors tested. The iR drop gradually decreases from LSG-MSC(4) through LSG-MSC(16), thus confirming the increase of power density of the micro-devices with an increasing number of interdigitated electrodes per unit area. 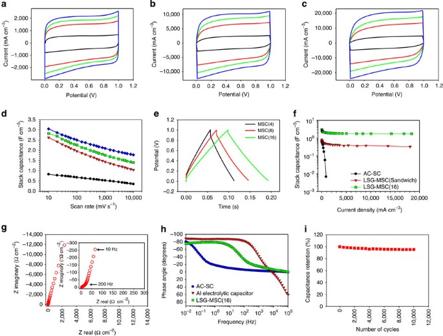Figure 3: Electrochemical performance of the LSG-MSC in PVA-H2SO4gelled electrolyte CV profiles of LSG-MSC in sandwich and interdigitated structures with 4, 8 and 16 electrodes at scan rates of (a) 1,000 mV s−1, (b) 5,000 mV s−1and (c) 10,000 mV s−1. (d) Evolution of the specific capacitance of the different supercapacitors as a function of the scan rate. Symbol key fora–d: sandwich (black), MSC(4) (red), MSC(8) (green) and MSC(16) (blue). (e) Galvanostatic charge/discharge curves of micro-supercapacitors based on interdigitated structures with 4, 8 and 16 electrodes, all operated at an ultrahigh current density of 1.68 × 104mA cm−3. (f) Volumetric stack capacitance of LSG-MSC in the sandwich and interdigitated structures as calculated from the charge/discharge curves at different current densities. Data for a commercial AC-SC are shown for comparison. (g) Complex plane plot of the impedance of a LSG-MSC(16) with a magnification of the high-frequency region is provided in the inset. (h) Impedance phase angle versus frequency for LSG-MSC(16) compared with commercial AC-SC and aluminium electrolytic capacitors. (i) The LSG-MSC(16) shows excellent stability, losing only about 4% of its initial capacitance over 10,000 cycles. Figure 3f shows the volumetric capacitance of the stack as a function of the current density for the LSG micro-supercapacitor for both the interdigitated and sandwich structures. For comparison, the data for a commercial activated carbon supercapacitor (AC-SC) obtained under the same dynamic conditions are also shown. Not only does the AC-SC exhibit lower capacitance, but its performance falls off very quickly at higher charge/discharge rates because of the limited diffusion of ions in the inner porous network of the activated carbon [11] , [24] . The surface of the LSG, on the other hand, is highly accessible to the electrolyte, with very little impediment to ion transport, thus providing high capacitance even when operated at ultrahigh charge/discharge rates (see Supplementary Fig. S9 for more details). For example, LSG-MSC(16) exhibits a stack capacitance of 3.05 F cm −3 at 16.8 mA cm −3 , and maintains 60% of this value when operated at an ultrahigh current density of 1.84 × 10 4 mA cm −3 , Fig. 3f . This is equivalent to the operation of the device at ~1100 A g −1 LSG/electrode , which is about 3 orders of magnitude higher than the normal discharge current densities used for testing traditional supercapacitors [2] , [3] . This corresponds to an areal capacitance that varies only slightly from 2.32 mF cm −2 at 16.8 mA cm −3 to 1.35 mF cm −2 at 1.84 × 10 4 mA cm −3 . This is superior to the values reported in the literature for EDLC micro-supercapacitors, with typical capacitance values of 0.4–2 mF cm −2 collected at much lower charge/discharge rates [2] , [4] , [25] . Figure 3: Electrochemical performance of the LSG-MSC in PVA-H 2 SO 4 gelled electrolyte CV profiles of LSG-MSC in sandwich and interdigitated structures with 4, 8 and 16 electrodes at scan rates of ( a ) 1,000 mV s −1 , ( b ) 5,000 mV s −1 and ( c ) 10,000 mV s −1 . ( d ) Evolution of the specific capacitance of the different supercapacitors as a function of the scan rate. Symbol key for a – d : sandwich (black), MSC(4) (red), MSC(8) (green) and MSC(16) (blue). ( e ) Galvanostatic charge/discharge curves of micro-supercapacitors based on interdigitated structures with 4, 8 and 16 electrodes, all operated at an ultrahigh current density of 1.68 × 10 4 mA cm −3 . ( f ) Volumetric stack capacitance of LSG-MSC in the sandwich and interdigitated structures as calculated from the charge/discharge curves at different current densities. Data for a commercial AC-SC are shown for comparison. ( g ) Complex plane plot of the impedance of a LSG-MSC(16) with a magnification of the high-frequency region is provided in the inset. ( h ) Impedance phase angle versus frequency for LSG-MSC(16) compared with commercial AC-SC and aluminium electrolytic capacitors. ( i ) The LSG-MSC(16) shows excellent stability, losing only about 4% of its initial capacitance over 10,000 cycles. Full size image Electrochemical impedance spectroscopy (EIS) further confirms the superior power performance of the LSG-MSC. The complex-plane plot of the impedance of LSG-MSC(16) shows pure capacitive behaviour even at high frequencies (200 Hz) owing to the highly accessible surface of the LSG, Fig. 3g . The equivalent series resistance obtained from the intercept of the plot on the real axis is only 3.6 Ω cm −2 , made manifest by the good ionic conductivity of the electrolyte and the low internal resistance of the microelectrodes. Remarkably, the LSG micro-supercapacitor shows superior frequency response with an extremely small relaxation time, Fig. 3h . Data from a commercial AC supercapacitor and an aluminium electrolytic capacitor are included for comparison. The RC time constant of LSG-MSC(16) was calculated to be 19 ms, in comparison with 10,000 ms for the commercial AC-SC and 1.1 ms for the electrolytic capacitor ( Supplementary Table S1 ). This extremely small time constant for the LSG-MSC(16) is very promising compared with previously reported values for planar micro-supercapacitors: activated carbon (700 ms) [2] , onion-like carbon (26 ms) [2] and graphene/CNT composite (4.8 ms) [3] . Furthermore, the LSG supercapacitors show excellent cycling stability, retaining 96% of the initial performance after 10,000 charge/discharge cycles. Bendable and twistable LSG-MSC Flexible electronics have recently attracted much attention because of their potential in providing cost-efficient solutions to large-area applications, such as roll-up displays and TVs, e- paper, smart sensors, transparent radio frequency identifications and even wearable electronics [26] . However, the fabrication of micro-supercapacitors on flexible substrates using current micro-fabrication techniques does not appear to be feasible. Attempts to fabricate micro-supercapacitors on flexible substrates using a number of printing and electrochemical techniques have also been reported [27] , [28] . However, none of these configurations have been shown to be suitable for flexible energy-storage devices. In fact, the performance durability of these devices has not been examined under any strain conditions such as bending or twisting. LSG-MSC are highly flexible and can be bent and twisted without affecting the structural integrity of the device, Fig. 4a (see also Supplementary Discussion ). To prove the durability of LSG-MSC for flexible energy storage, we tested their electrochemical performance under constant strain. 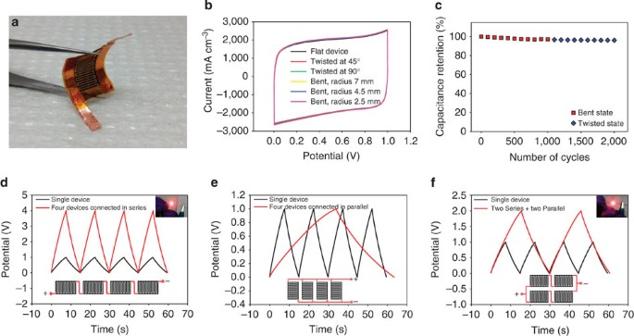Figure 4: Behaviour of LSG-MSC under mechanical stress and in series/parallel combinations (a) A photograph of LSG-MSC(16) bent with a tweezers demonstrates the flexibility of the micro-device. (b) Bending/twisting the device has almost no effect on its performance, as can be seen from these CVs collected under different bending and twisting conditions at 1,000 mV s−1. (c) Performance durability of the micro-device when tested under bending and twisting conditions. The device retains ~97% of its initial capacitance after 1,000 cycles under the bent state, followed by another 1,000 cycles under the twisted state. Galvanostatic charge/discharge curves for four tandem micro-supercapacitors connected (d) in series, (e) in parallel and (f) in a combination of series and parallel. A single device is shown for comparison. Both the tandem devices and the single device were operated at the same charge/discharge current. (Insets) the tandem micro-supercapacitor can be used to power a light-emitting diode (LED). Figure 4b shows the CV performance of the micro-supercapacitor with different bending and twisting conditions at 1,000 mV s −1 . The micro-supercapacitor shows exceptional electrochemical stability regardless of the degree of bending or twisting, indicating excellent mechanical stability. The flexibility endurance of the device was tested while keeping the device under the bent or twisted state, Fig. 4c . Remarkably, the capacitance was reversibly maintained with 97% retention of the initial capacitance after 2,000 cycles. This superior performance makes LSG-MSC promising for flexible micro-electronics. Figure 4: Behaviour of LSG-MSC under mechanical stress and in series/parallel combinations ( a ) A photograph of LSG-MSC(16) bent with a tweezers demonstrates the flexibility of the micro-device. ( b ) Bending/twisting the device has almost no effect on its performance, as can be seen from these CVs collected under different bending and twisting conditions at 1,000 mV s −1 . ( c ) Performance durability of the micro-device when tested under bending and twisting conditions. The device retains ~97% of its initial capacitance after 1,000 cycles under the bent state, followed by another 1,000 cycles under the twisted state. Galvanostatic charge/discharge curves for four tandem micro-supercapacitors connected ( d ) in series, ( e ) in parallel and ( f ) in a combination of series and parallel. A single device is shown for comparison. Both the tandem devices and the single device were operated at the same charge/discharge current. (Insets) the tandem micro-supercapacitor can be used to power a light-emitting diode (LED). Full size image In general, the total energy that can be stored in a single supercapacitor is too low for most practical applications. Thus, depending on the application, supercapacitors need to be connected together in series and/or parallel combinations, just as batteries are, to form a ‘bank’ with a specific voltage and capacitance rating. The adaptability of LSG-MSC for serial/parallel combinations is demonstrated by connecting four devices together both in series and in parallel configurations, Fig. 4d–f . The tandem LSG-MSC exhibit a very good control over the operating voltage window and capacity, thus enabling them to be considered for practical applications. Similar to the individual micro-supercapacitors, the tandem devices exhibit essentially ideal triangular charge/discharge curves with a minute voltage drop, which again indicates excellent capacitive properties with minimal internal resistance. It is worth noting that this exceptional performance has been achieved without using a voltage balance, which is often needed with series connections to prevent any cell from going into over-voltage. Ionogels—devices with high energy and power densities Previous research attempts to design supercapacitors in the all-solid-state form have focused mainly on using aqueous hydrogel-polymer electrolytes. Unfortunately, the operating voltage range of these devices barely exceeds 1 V, making them non-functional for many applications. Unlike water-based electrolytes, ionic liquids (ILs) provide an attractive alternative to these conventional electrolytes owing to their wide electrochemical window and high ionic conductivity, as well as good thermal stability and non-volatility [29] . These interesting properties of ILs can be hybridized with another solid component (for example, polymer, silica, and so on) to form gel-like electrolytes called ionogels [30] . The combination of a solid matrix with ILs preserve the main properties of ILs, while allowing easy shaping of the device without having the intrinsic leakage problems of liquid electrolytes that limit their flexible operation. Although promising, the integration of ionogels into all-solid-state micro-supercapacitors has not yet been demonstrated. Here, we mixed together fumed silica (FS) nanopowder with the IL 1-butyl-3-methylimidazolium bis(trifluoromethylsulfonyl)imide to form a clear viscous (FS-IL) ionogel, Fig. 5a (see also Supplementary Fig. S10 ). The ionogel was integrated into an all-solid-state device, and its electrochemical performance is shown in Supplementary Fig. S11 . Interestingly, the device demonstrates ultrahigh charge/discharge rates comparable to those with PVA-H 2 SO 4 hydrogel electrolyte, but the device can now be operated at a larger potential window of 2.5 V, Supplementary Figs S11 and S12 . The almost ideal CV profiles and triangular charge/discharge curves at ultrafast charge/discharge rates verify good EDLC behaviour. The LSG-MSC(16) achieved a stack capacitance of 2.35 F cm −3 at a current density of 16.8 mA cm −3 . When operated at an ultrafast charge/discharge current density of 1.84 × 10 4 mA cm −3 , the capacitance of the device drops only slightly to 1.40 F cm −3 . As the energy density increases with the square of the operating potential window, the micro-supercapacitor using an FS-IL ionogel promises an order of magnitude higher energy density. Furthermore, the high thermal stability of ILs eliminates the fire hazards associated with commercial supercapacitors. Finally, the micro-supercapacitor shows excellent cycling stability; the capacitance remains unchanged after more than 30,000 charge/discharge cycles. 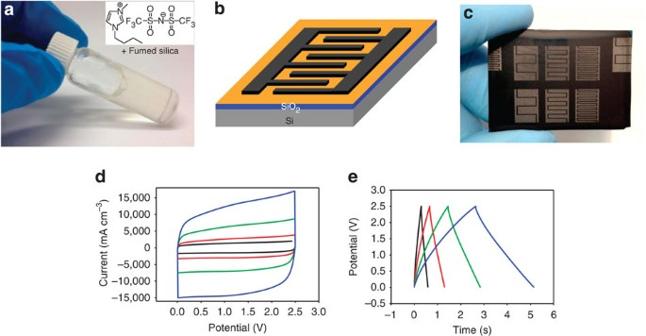Figure 5: Fabrication and characterization of LSG-MSC on a chip LightScribe can be used to produce LSG-MSC directly on a chip that contains integrated circuits, which they can then power. (a) An ionogel electrolyte was used in the assembly of the device. It is prepared by mixing together the ionic liquid 1-butyl-3-methylimidazolium bis(trifluoromethylsulfonyl)imide with fumed silica nanopowder. (b) Schematic of the device; (c) Photograph of the micro-devices. (d) CV profile of LSG-MSC(16) at various scan rates, from low to high: 1000 (black), 2000 (red), 5000 (green) and 10000 (blue) mV s−1. (e) Galvanostatic charge/discharge curves of LSG-MSC(16) collected at different current densities: 1.06 × 104(black), 5.05 × 103(red), 2.42 × 103(green) and 1.38 × 103(blue) mA cm−3. Figure 5: Fabrication and characterization of LSG-MSC on a chip LightScribe can be used to produce LSG-MSC directly on a chip that contains integrated circuits, which they can then power. ( a ) An ionogel electrolyte was used in the assembly of the device. It is prepared by mixing together the ionic liquid 1-butyl-3-methylimidazolium bis(trifluoromethylsulfonyl)imide with fumed silica nanopowder. ( b ) Schematic of the device; ( c ) Photograph of the micro-devices. ( d ) CV profile of LSG-MSC(16) at various scan rates, from low to high: 1000 (black), 2000 (red), 5000 (green) and 10000 (blue) mV s −1 . ( e ) Galvanostatic charge/discharge curves of LSG-MSC(16) collected at different current densities: 1.06 × 10 4 (black), 5.05 × 10 3 (red), 2.42 × 10 3 (green) and 1.38 × 10 3 (blue) mA cm −3 . Full size image Direct fabrication of an LSG-MSC on a chip Current trends for developing miniaturized electronic devices place emphasis on achieving performance levels generally associated with integrated circuits. Here, we demonstrate an on-chip micro-supercapacitor that can be integrated with MEMS devices and CMOS in a single chip using the LightScribe direct writing technique. The structure of the device is schematically illustrated in Fig. 5b , with an ionogel used as the electrolyte. The device was fabricated using the same process described earlier, except for the plastic substrate that has been replaced with an oxidized silicon wafer, Fig. 5c . Figure 5d shows that the device reveals superior electrochemical performance with ultrahigh power, comparable to that demonstrated on the flexible substrate. This technique may thus present a low-cost and scalable solution for on-chip self-powered systems. Low leakage current and slow self-discharge rate Charged supercapacitors, such as charged batteries, are in a state of high free energy relative to that of the discharged state, and thus there is a thermodynamic driving force for them to self-discharge [31] . The self-discharge behaviour of supercapacitors is a matter of major practical significance in their operation and the types of function they may be required to fulfil. During self-discharge, a small amount of leakage current will cause the voltage decay of a charged supercapacitor over time. The leakage current can be measured by applying a rated DC voltage to the supercapacitor and measuring the current required to maintain that voltage. Typically, this is done using the voltage at which the supercapacitor is operated, V max . The results are presented in Fig. 6a which also include the data for two commercially available supercapacitors, all tested under the same dynamic conditions. The results show that the LSG micro-supercapacitor exhibits an ultra-small leakage current of <150 nA after 12 h compared with ~5 μA for both of the commercial supercapacitors. With its low leakage current, LSG-MSC could be integrated with energy harvesters to create efficient self-powered systems. 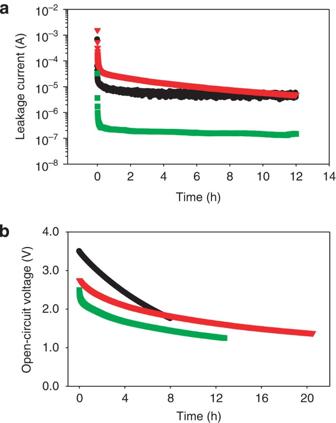Figure 6: Testing the self-discharge rate of LSG-MSC (a) Leakage current measurement of an LSG micro-supercapacitor (with 16 interdigitated electrodes) and two commercially available supercapacitors. A DC voltage (the voltage at which the supercapacitor is operated,Vmax) was applied across the capacitor; the current required to retain that voltage was measured over a period of 12 h. (b) Self-discharge curves of the respective supercapacitors obtained immediately after precharging toVmaxin the previous test. This involves measuring the open-circuit voltage across the supercapacitors betweenVmaxand ½Vmaxversus the course of time. This involves 3.5 V/25 mF commercial supercapacitor (black), 2.75 V/44 mF commercial supercapacitor (red) and LSG micro-supercapacitor assembled using ionogel electrolyte (green). Figure 6: Testing the self-discharge rate of LSG-MSC ( a ) Leakage current measurement of an LSG micro-supercapacitor (with 16 interdigitated electrodes) and two commercially available supercapacitors. A DC voltage (the voltage at which the supercapacitor is operated, V max ) was applied across the capacitor; the current required to retain that voltage was measured over a period of 12 h. ( b ) Self-discharge curves of the respective supercapacitors obtained immediately after precharging to V max in the previous test. This involves measuring the open-circuit voltage across the supercapacitors between V max and ½ V max versus the course of time. This involves 3.5 V/25 mF commercial supercapacitor (black), 2.75 V/44 mF commercial supercapacitor (red) and LSG micro-supercapacitor assembled using ionogel electrolyte (green). Full size image The self-discharge curves obtained immediately after precharging to V max in the previous test are shown in Fig. 6b . Basically, the voltage difference between the two terminals of the supercapacitor is recorded on an open circuit as a function of time. Normally, most supercapacitors are operated in the range of V max to approximately ½ V max (ref. 32 ). Thus, the time required for the voltage across the supercapacitor to change from V max to ½ V max was measured for all of the tested supercapacitors. The results show that the LSG micro-supercapacitor self-discharges in 13 h, a value comparable to those of commercial supercapacitors, with self-discharge rates of 8 h and 21 h. This fine performance for the LSG-MSC shows promise for practical applications. 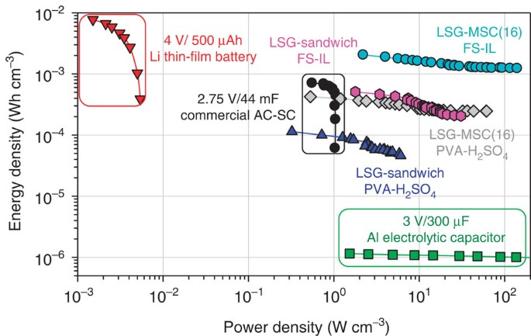Figure 7: Energy and power densities of LSG-MSCs compared with commercially available energy-storage systems LSG-MSCs exhibit ultrahigh power and energy densities compared with a commercially available AC-SC, an aluminium electrolytic capacitor and a lithium thin-film battery. LSG micro-devices can deliver ultrahigh power density comparable to those of an aluminium electrolytic capacitor, while providing three orders of magnitude higher energy density. Data for the Li battery are reproduced from ref.2. Figure 7 shows a Ragone plot comparing the performance of LSG-MSC with different energy-storage devices designed for high-power microelectronics (see Supplementary Methods ). The plot shows the volumetric energy density and power density of the stack for all the devices tested. It reveals a significant increase in the supercapacitor performance when scaling down the electrode dimensions to the micro-scale. For example, the interdigitated micro-supercapacitors deliver more energy and power than their sandwich counterparts both in the hydrogel-polymer and ionogel electrolytes. Remarkably, compared with the AC supercapacitor, the LSG micro-device exhibits 3 times more energy and ~200 times more power. Furthermore, the LSG-MSC demonstrates power densities comparable to those of the aluminium electrolytic capacitor, while providing more than 3 orders of magnitude higher energy density. Although Li-ion batteries can provide high energy density, they have limited power performance that is 4 orders of magnitude lower than the LSG-MSC. This superior energy and power performance of the LSG-MSC should enable them to compete with micro-batteries and electrolytic capacitors in a variety of applications. See also a comparison between LSG-MSC and the state-of-the-art ultrahigh-power micro-supercapacitors reported in the literature, Supplementary Table S2 . Further miniaturization of the width of the micro-electrodes and the space between them would reduce the ionic diffusion pathway, thus leading to micro-supercapacitors with higher power density. Figure 7: Energy and power densities of LSG-MSCs compared with commercially available energy-storage systems LSG-MSCs exhibit ultrahigh power and energy densities compared with a commercially available AC-SC, an aluminium electrolytic capacitor and a lithium thin-film battery. LSG micro-devices can deliver ultrahigh power density comparable to those of an aluminium electrolytic capacitor, while providing three orders of magnitude higher energy density. Data for the Li battery are reproduced from ref. 2 . Full size image The single-step fabrication technique described here obviates the need for time consuming and labour-intensive lithography, while enhancing the yield of the process and the functionality of the micro-devices produced. Remarkably, this technique allows for the fabrication of micro-devices without the use of organic binders, conductive additives or polymer separators that are often needed in commercial supercapacitors, thus leading to improved performance because of the ease with which ions can access the active material. The combination of the microscale design of the device with LSG whose surface is fully accessible to electrolyte ions is responsible for the high-power/energy performance of the LSG-MSC. They combine the power density of electrolytic capacitors with the energy density of micro-batteries, which could have a significant impact on high-power microelectronics. These findings also provide a solution to microscale energy storage in numerous areas in which electrolytic capacitors cannot provide sufficient volumetric energy density. Furthermore, LSG-MSC show excellent cycling stability. This is very important when compared with micro-batteries whose finite lifetime could be a major problem when they have to be embedded in permanent structures, such as biomedical implants, active radio frequency identification tags and embedded micro-sensors where no maintenance or replacement is possible. As these micro-supercapacitors can be directly integrated on-chip, they may help to better extract the energy from solar, mechanical and thermal sources and thus make more efficient self-powered systems [33] . They could also be fabricated on the backside of solar cells in both portable devices and rooftop installations, to store power generated during the day for use after sundown, and thus may help provide electricity around the clock where connection to the grid is not possible. Other applications could arise that take advantage of the flexible nature of the substrates, such as electronics embedded into clothing, large-area flexible displays and roll-up portable displays [23] , [34] . Fabrication of LSG-MSC LSG-MSCs were produced by the direct writing of graphene patterns on GO films using a consumer-grade LightScribe DVD burner. Briefly, GO was synthesized using a modified Hummer’s method [35] , and aqueous dispersions of GO with the appropriate concentration (2.7 mg ml −1 ) were made. A sheet of plastic, polyethylene terephthalate (PET), was glued to the surface of a LightScribe DVD media disc. A volume of 16 ml of GO solution was then drop-cast on PET and allowed to dry overnight under ambient conditions. The GO-coated DVD disc was then inserted into the DVD optical drive for laser patterning. Interdigitated micro-patterns designed using regular computer software were directly LightScribed onto the GO film. This LightScribing process converts the golden-brown insulating GO into black highly conducting LSG patterns at precise locations. With the laser precision, the drive renders the computer-designed patterns onto the GO film to produce the graphene micro-patterns in about 20 min. The LSG micro-patterns were directly used as micro-supercapacitors after receiving an electrolyte overcoat. Here, LSG serves as both the active electrode material and the current collector. For electrochemical characterization of the micro-devices, copper tape was applied to the electrode edges to ensure good electrical contact between the LSG devices and the electrochemical workstation. For better current collection, the copper tape was glued to the electrodes using silver paint. The interdigitated area is defined with polyimide (Kapton) tape to protect the contact pad from the electrolyte. The electrolyte was drop-cast on the active interdigitated electrode area, and left under ambient conditions for 3 h to ensure that the electrolyte completely wets the electrode and to allow for evaporation of any excess water. LSG micro-devices can be made on virtually any substrate. For example, we made devices on silicon wafers to demonstrate the potential of the technique for the direct fabrication of LSG-MSCs for the next generation of CMOS applications. Si/SiO 2 (500 nm) wafers of the appropriate size were glued to the surface of the DVD media disc and coated with a GO solution as previously described and then LightScribed in the drive to produce the micro-devices. Characterization and measurements The microstructures of GO and LSG micro-devices were investigated by means of field emission scanning electron microscopy (JEOL 6700) and optical microscopy (Zeiss Axiotech 100). Electrical measurements (I–V curves) were carried out on a VersaSTAT3 electrochemical workstation (using a two-electrode setup) by measuring the current produced at different gate voltages (from −1 to +1) with a potentiostatic technique. To prevent the graphene network from being damaged by the probes, two contact electrodes were first made by carefully painting a layer of silver (SPI supplies, Pennsylvania, USA) on the LSG film. Ten measurements were performed on different areas of the film to ensure reproducibility. The thicknesses of the different components of the device were measured using cross-sectional scanning electron microscopy and a Dektak 6 profilometer. Conductivity values were calculated from the slopes of the I–V curves and the thickness of each film. The electrochemical performances of the LSG-MSC were investigated by CV, galvanostatic charge/discharge tests and EIS. CV and charge/discharge testing were performed on a VersaSTAT3 electrochemical workstation (Princeton Applied Research, USA). EIS measurements were recorded on a Solartron electrochemical workstation (Solartron Analytical, Oak Ridge, TN) over a frequency range of 100 kHz to 10 MHz with an amplitude of 10 mV at the open-circuit potential. The characterization experiments of the devices using PVA-H 2 SO 4 were performed in air, whereas those made with ionogel electrolyte were fully characterized in an argon-filled glove bag. All experiments were performed at room temperature. Calculations of the specific capacitance and the energy and power densities are discussed in detail in the Supplementary Methods . How to cite this article: El-Kady, MF. et al. Scalable fabrication of high-power graphene micro-supercapacitors for flexible and on-chip energy storage. Nat. Commun. 4:1475 doi: 10.1038/ncomms2446 (2013).